Topological protection of bound states against the hybridization Topological invariants are conventionally known to be responsible for protection of extended states against disorder. A prominent example is the presence of topologically protected extended states in two-dimensional quantum Hall systems as well as on the surface of three-dimensional topological insulators. Here we introduce a new concept that is distinct from such cases—the topological protection of bound states against hybridization. This situation is shown to be realizable in a two-dimensional quantum Hall insulator put on a three-dimensional trivial insulator. In such a configuration, there exist topologically protected bound states, localized along the normal direction of two-dimensional plane, in spite of hybridization with the continuum of extended states. The one-dimensional edge states are also localized along the same direction as long as their energies are within the band gap. This finding demonstrates the dual role of topological invariants, as they can also protect bound states against hybridization in a continuum. Bound states of electrons in solids offer many intriguing phenomena. For instance, localized states are common in the presence of impurities, and donor and acceptor levels are the main issue in semiconductor physics and technology. Bound states can also appear in clean systems and their existence attributes to topological origins in many cases. Solitons in polyacetylene are associated with the midgap states, which emerge owing to topological reason, and control the electric, magnetic and optical properties of the system [1] , [2] , [3] . One-dimensional (1D) conducting channels at the edge of the quantum Hall and quantum spin Hall systems are another example of bound states in clean systems, which determines the low-energy transport phenomena [4] , [5] , [6] , [7] , [8] . Bulk-edge correspondence guarantees the existence of these edge channels, that is, they are protected by the gap and the non-trivial topology of the bulk states [9] , [10] . A recent remarkable advance in the study of three-dimensional (3D) topological insulators, which support the helical Dirac fermion on the surface of the sample, provides another example of bound states belonging to the same category [11] , [12] , [13] , [14] . A common feature of all these cases is that the energy of the bound state is within the energy gap of the extended states. The extended states constitute the continuum of the density of states even though the disorder potential makes the crystal momentum k ill-defined. Usually, the extent of the localized state is determined by the inverse of the energy separation between the localized level and the edge of the continuum. In general, it is believed that no state can be localised within this continuum owing to the hybridization with the extended states, as discussed in detail in Supplementary Note 1 , although there are several proposals for creating a bound state in a continuum by engineering the effective coupling between the discrete level and the continuum states [15] , [16] , [17] . This fact is the essential reason for the existence of the mobility edge, E c in disordered systems [18] . Namely, there is a critical energy, E c , separating the extended and localized states. In this paper, we study the electronic states of the two-dimensional (2D) quantum Hall insulator (QHI) on the substrate of a topologically trivial 3D normal insulator (NI). One remarkable discovery through this study is that there are bound states even in the continuum of the Bloch states of the substrate. The hybridization with the Bloch states does not destroy the localization of some bulk states of the QHI along the z direction perpendicular to the surface. This is the first example for the existence of bound states within the continuum of extended states, which are protected by the topology. Structure of the system A schematic diagram describing the structure of the system is shown in Fig. 1a . We first consider a 2D QHI supporting 1D chiral edge states (CESs) on its boundary and a fully gapped 3D NI separately and then put the QHI on the top surface of the 3D NI. As shown in Fig. 1b , the typical band structure of the coupled system is composed of three inequivalent parts, that is, the 3D continuum states from the 3D NI and the 2D bulk, and 1D CES from the QHI. There are two main questions to address here. One is whether the 2D bulk states of the QHI are exponentially localized near the top surface layer or they are spread out along the z direction when the 2D QHI and 3D NI are strongly hybridized, especially, when the 2D QHI bands are fully buried in the continuum of the 3D NI bands. The other is what the spatial distribution of the 1D CES is along the z direction in this case. These two issues are closely related because if the 2D states are extended and diluted along the z direction, it is natural to expect the CES to be extended and diluted, as well. As for the fate of 1D chiral states coupled to a continuum, it is reminiscent of a recent theoretical work demonstrating the stability of the helical surface states of topological insulators against the hybridization with additional non-topological bulk metallic states [19] . However, it is worth noting that the stability of 1D chiral states in our system is essentially a new issue because when the 2D QHI is coupled to a 3D substrate, even the stability of the 2D QHI bulk state itself supporting the boundary chiral fermions is not guaranteed. 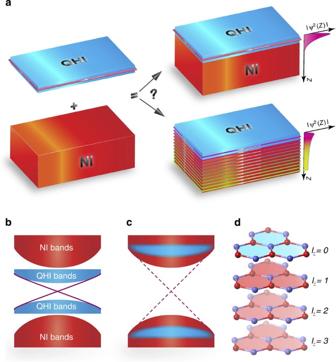Figure 1: Geometry and energy band diagram of the heterostructure composed of 2D QHI and 3D NI. (a) A schematic diagram showing the structure of the system. A 2D QHI with 1D CES is attached on the top surface of a 3D NI. One main question is whether the 1D CES is localized or extended along thezdirection when 2D QHI and 3D NI are coupled. The typical energy spectra of the full heterostructure in the momentum space are shown in (b) and (c). The NI bands (QHI bands) are the states coming from NI (QHI) and the dispersion in the gap corresponds to the (possible) 1D edge channel. (d) A hexagonal lattice model composed of 2D honeycomb lattices stacked along thezdirection. The QHI on the top layer () is coupled to the 3D NI composed of stacked 2D trivial insulator layers (). Figure 1: Geometry and energy band diagram of the heterostructure composed of 2D QHI and 3D NI. ( a ) A schematic diagram showing the structure of the system. A 2D QHI with 1D CES is attached on the top surface of a 3D NI. One main question is whether the 1D CES is localized or extended along the z direction when 2D QHI and 3D NI are coupled. The typical energy spectra of the full heterostructure in the momentum space are shown in ( b ) and ( c ). The NI bands (QHI bands) are the states coming from NI (QHI) and the dispersion in the gap corresponds to the (possible) 1D edge channel. ( d ) A hexagonal lattice model composed of 2D honeycomb lattices stacked along the z direction. The QHI on the top layer ( ) is coupled to the 3D NI composed of stacked 2D trivial insulator layers ( ). Full size image To understand the effects of the hybridization between the 2D QHI and the 3D substrate, we first study numerically a hexagonal lattice system composed of stacked 2D honeycomb lattices as shown in Fig. 1d . Here, we treat the 3D NI as a system composed of coupled 2D layers stacked along the z direction, where each layer is labelled with the index . The top layer labelled with represents a 2D QHI, which is coupled to the 3D NI through the inter-layer hopping transfer between nearest neighbours. The detailed description of the lattice Hamiltonian is given in the Methods section. Localized state in a continnum In Fig. 2 , we plot the energy dispersion along the k x axis and the localization profile of the system. From Fig. 2a to Fig. 2c , the energy gap of the 3D NI is gradually decreased, while the other parameters of the QHI are fixed. Also, layer-resolved wave function amplitudes are shown in each panel. When the QHI bands are fully separated from the continuum as in Fig. 2a , the wave functions of the QHI are almost completely localized in the first two layers. On the other hand, Fig. 2b shows that when the QHI and NI bands overlap in a finite interval, the parts separated from (touching) the continuum are localized (extended). However, surprisingly, the bound states still exist even when the QHI bands are fully buried in the continuum as shown in Fig. 2c . In Fig. 2c , there is a window near the corner of the Brillouin zone, marked with dotted circles, in which bound states exist within the continuum states. Especially, in this case, the states at this corner of the Brillouin zone are completely localized, therefore their wave function amplitudes become zero within the accuracy of our numerics for . In Fig. 2g–h , we plot the dependence of the squared wave function amplitude of the localized states at the two corners of the hexagonal Brillouin zone. To compare the wave function spreading at the two corners on the k x axis, we have changed the strength of the inter-layer coupling between the top and its neighbouring layers relative to the inter-layer coupling inside the 3D NI, which is defined as P . For given P and the momentum, we have picked one state, among the eigenstates, which has the highest wave function amplitude on the top layer. When the top layer is decoupled from the rest of the system, that is, when P =0, there are completely localized states at both corners. However, when P increases to P =0.5 and finally to P =1, the state localized at the left corner spreads rapidly along the z direction ( Fig. 2h ) while the localized state on the right corner survives without any spreading of the wave function amplitude ( Fig. 2g ). The distribution of localized states in the Brillouin zone is reflected in Fig. 2d–f in which the squared wave function amplitudes of the localized states on the top layer ( ) are plotted. 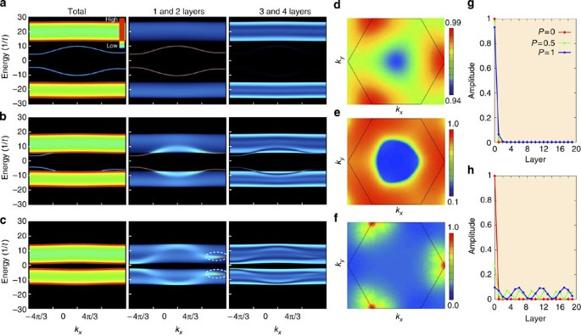Figure 2: Energy dispersion and distribution of localized states of 2D QHI bulk bands in a continuum. Energy dispersion and the distribution of localized 2D bulk states of the coupled system composed of honeycomb layers stacked along thedirection. Bulk band structure of the system alongky=0 is shown in (a–c) where the NI bands and QHI bands are not touching, partially ovarlapped and fully overlapped, respectively. From (a–c), the energy gap of the NI band is progressively reduced while the spectrum of the QHI band remains the same. In each panel, the layer-resolved wave function amplitudes ofare shown. Hereis then-th eigenfunction at the momentum. The localized bound states are almost completely confined within the first two layers. The dotted circles on the second figure from the left in the panel (c) indicate the localized bound states existing within the continuum states. In (d–f), we have picked up one state among all the eigenstates at each, which has the maximum value of, and then the resulting squared amplitude ofis plotted over the entire Brillouin zone for systems corresponding to (a–c), respectively. Finally, in (g,h), thedependence of the squared wave function amplitudesof the localized state is plotted for(g) and for(h). Here we have varied the strength of the inter-layer coupling between the top and its neighbouring layers relative to the inter-layer coupling inside the 3D NI, which is defined asP. For fixedPand, we have picked the eigenfunction that has the highest amplitude on the top layer and plotted itsdependence. Figure 2: Energy dispersion and distribution of localized states of 2D QHI bulk bands in a continuum. Energy dispersion and the distribution of localized 2D bulk states of the coupled system composed of honeycomb layers stacked along the direction. Bulk band structure of the system along k y =0 is shown in ( a – c ) where the NI bands and QHI bands are not touching, partially ovarlapped and fully overlapped, respectively. From ( a – c ), the energy gap of the NI band is progressively reduced while the spectrum of the QHI band remains the same. In each panel, the layer-resolved wave function amplitudes of are shown. Here is the n -th eigenfunction at the momentum . The localized bound states are almost completely confined within the first two layers. The dotted circles on the second figure from the left in the panel ( c ) indicate the localized bound states existing within the continuum states. In ( d – f ), we have picked up one state among all the eigenstates at each , which has the maximum value of , and then the resulting squared amplitude of is plotted over the entire Brillouin zone for systems corresponding to ( a – c ), respectively. Finally, in ( g , h ), the dependence of the squared wave function amplitudes of the localized state is plotted for ( g ) and for ( h ). Here we have varied the strength of the inter-layer coupling between the top and its neighbouring layers relative to the inter-layer coupling inside the 3D NI, which is defined as P . For fixed P and , we have picked the eigenfunction that has the highest amplitude on the top layer and plotted its dependence. Full size image Topological stability of the localized state in a continuum In fact, remarkably, the bound state in a continuum has topological stability. Namely, the bound state always exists in the Brillouin zone and cannot be removed by applying small perturbations. It is to be noted that, as shown in Fig. 2 , the lattice model we have considered has a threefold rotational symmetry ( C 3 ) while all the other point group symmetries are explicitly broken. To rule out the symmetry protection of the localized state at the corner of the Brillouin zone, we have introduced a term breaking C 3 symmetry and confirmed that the localized state survives even when all the point group symmetries of the system are completely broken. In addition, the stability of such localized bound states is further supported by additional numerical data demonstrating that localized bound states always exist irrespective of the lattice structure and the nature of the inter-layer coupling between the 2D QHI and 3D NI. The detailed information about the additional numerical results is provided in Supplementary Fig. S1 and Supplementary Note 2 . The topological stability of the localized state can be understood in the following way. The minimal Hamiltonian for the 2D QHI and 3D NI, which describes one conduction band and one valence band with a finite gap between them, can be written as and where are Pauli matrices. Here is a function of the in-plane momentum while H 0 and depend on the three momenta ( k x , k y , k z ). Considering the coupling between the 2D QHI and 3D NI, in general, the retarded Green’s function for the effective 2D QHI can be written as where when is within the 3D NI bands and otherwise. In equation (1), the unit vector , in which sign ( sign) corresponds to the case of lying within the 3D bulk conduction (valence) band. It is to be noted that here and depend on . The k z dependence of is replaced by the dependence through the k z integration in the self-energy correction. Also the minor correction from the real part of the self-energy is neglected; however, it does not affect the generality of the conclusion. The detailed derivation procedures to obtain G R can be found in Supplementary Note 3 . Then immediately leads to . Namely, when the unit vector is parallel (anti-parallel) to , a Delta function singularity of G R appears at ( ), which corresponds to the bound state and the localization along the z direction. Let us discuss about the physical meaning of the condition . In the case of the QHI with the Hamiltonian , the unit vector forms a skyrmion configuration in the 2D momentum space and the wrapping number (or the skyrmion number) of over the first Brillouin zone is equal to the Chern number of the QHI [20] . On the other hand, as stems from the Hamiltonian of the 3D NI, generally, cannot have non-zero skyrmion number. Namely, the unit vector describes a topologically trivial configuration. 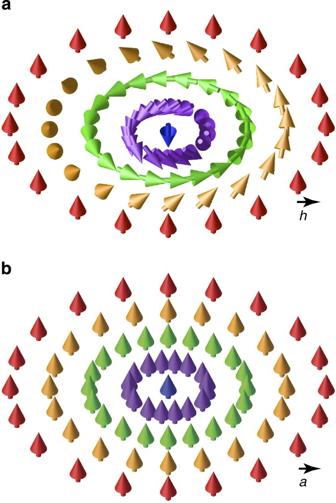Figure 3: Topological origin of bulk localization. Schematic figures showing the topological structure of the unit vectorsandin a 2D space. (a)forms a skyrmion configuration with the unit Pontryagin number while (b)makes a topologically trivial structure.andare parallel (anti-parallel) at the boundary (at the centre). Figure 3 shows the orientations of and , in which forms a skyrmion configuration with the unit Pontryagin number. It is to be noted that there are two special points, one at the centre and the other at the boundary of the circle, where or is satisfied, respectively. One of the two special points satisfies the condition for bulk localization, either in the conduction band or in the valence band. Therefore, there should be at least one localized 2D bulk state in each of the conduction and valence bands. The key ingredient leading to the topological protection of the localized bound state is that the points satisfying cannot be removed as long as and describe topologically inequivalent configurations. In general, the minimum number of completely localized states buried in a continuum band is given by where is the skyrmion number (or Chern number) covered by the unit vector . Figure 3: Topological origin of bulk localization. Schematic figures showing the topological structure of the unit vectors and in a 2D space. ( a ) forms a skyrmion configuration with the unit Pontryagin number while ( b ) makes a topologically trivial structure. and are parallel (anti-parallel) at the boundary (at the centre). Full size image Localization of 1D CESs Now we turn to the localization problem of the 1D CES. To observe the 1D CES numerically, we have introduced boundaries with zigzag-type edges on each honeycomb layer. It is confirmed that in all three cases corresponding to Fig. 2a–c , the 1D CES exists and is localized on the top few layers. Especially, as shown in Figs 2c , 4 , it is valid even when the QHI bands are fully buried in the continuum, hence a part of the 1D CES is hybridized with the continuum states. However, the hybridization with the continuum states does not simply destroy the 1D CES but instead the 1D CES is pushed away from the overlapping region into the bulk gap, which is consistent with the recent theory proposed by Bergman and Rafael [19] . The crucial point is that the existence of in-gap states is solely determined by the topology of H QHI . Moreover, once the CES exists, the fact that it is in the gap guarantees its localization along the z direction even if QHI bands are coupled to the continuum states. The detailed proof is given in Supplementary Note 4 . Therefore, as long as the gap between the conduction and valence bands of the QHI is not fully buried in the 3D continuum, the 1D CES should exist and be localized. 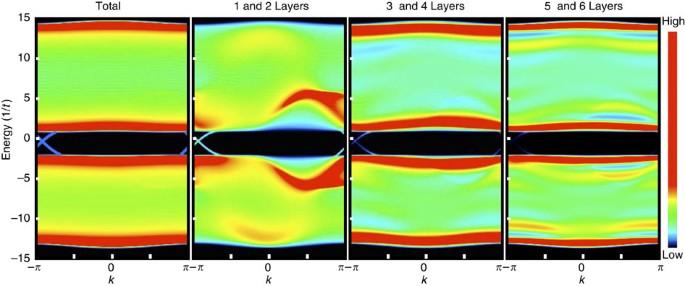Figure 4: Localization of 1D CES. Energy dispersion and layer-resolved wave function amplitudes of the finite size system corresponding toFig. 2c. To obtain the 1D chiral edge spectrum, we introduce two parallel zigzag edges in each honeycomb layer and stack the corresponding strip structures along thezaxis. Then the resulting system possesses two parallel surfaces whose surface normal direction is perpendicular to thezaxis. Figure 4: Localization of 1D CES. Energy dispersion and layer-resolved wave function amplitudes of the finite size system corresponding to Fig. 2c . To obtain the 1D chiral edge spectrum, we introduce two parallel zigzag edges in each honeycomb layer and stack the corresponding strip structures along the z axis. Then the resulting system possesses two parallel surfaces whose surface normal direction is perpendicular to the z axis. Full size image Extension to general cases The topological protection of the localized bound states against hybridization is a phenomenon that is valid in more general situations beyond the simple two-band model description considered up to now. Here, we provide additional numerical data supporting the generality of our theory. To construct general lattice models, we have modified the in-plane dispersion in the Hamiltonian of the 3D NI to lift its similarity to the Hamiltonian of the 2D QHI. The detailed structure of the modified Hamiltonian describing the 3D NI is shown in the Methods section. Let us discuss about the extension to multiband systems. For simplicity, we construct 2D four-band models attached to the two-band 3D NI. To distinguish the different Chern number distribution between the four bands on the top layer of the heterostructure, we use the following notation of C ≡[ C 1 , C 2 , C 3 , C 4 ] where C i indicates the Chern number of the i -th band. Here, the four bands are aligned in decreasing order of energy from the band 1 with the highest energy to the band 4 with the lowest energy. We first consider the case of C =[0,0,−1,+1]. Here, the two high (low)-energy bands are buried in the conduction (valence) band continuum of the 3D NI. From the 2D distribution of the states localized along the z direction as shown in the two right panels of Fig. 5a , we can clearly see the different degrees of localization between the topologically trivial bands and non-trivial bands buried in a continuum. This is also supported by the layer-resolved wave function amplitudes. Interestingly, even when the two 2D bands with opposite Chern numbers are buried in a single continuum band, so that the gap between the 2D bands is filled with continuum states, each of the 2D bands supports completely localized bulk states separately. This shows the fact that the number of localized 2D bulk states is solely determined by the Chern number difference between the 2D bulk band and the effective 2D band of the 3D NI, which is consistent with the conclusion based on the Green’s function analysis given above. On the other hand, as for the localization of the 1D CES, the existence of the band gap between the 2D bands supporting the CES is crucial. From the numerical analysis of the edge spectrum, it is confirmed that there is no 1D CES localized along the z direction in this case. We also have considered other model systems such as C =[−1,0,+1,0] ( Fig. 5b ), C =[0,−1,+1,0] ( Fig. 5c ), C =[−1,−1,+1,+1] ( Fig. 5d ) and C =[−1,+1,+1,−1] ( Fig. 5e ) cases. All of them support the same conclusion that the localization of the 2D bulk state is entirely determined by the Chern number of the 2D band buried in the continuum states of the topologically trivial 3D NI. However, the existence of the band gap is required for the localization property of the 1D CES in addition to the topological property of the 2D bulk states supporting the 1D CES. 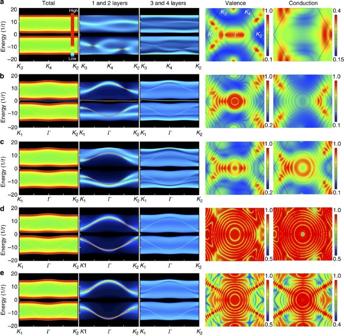Figure 5: Energy dispersion and distribution of localized states of 2D four-band QHI bulk bands in a continuum of the 3D NI. Energy dispersion and localization profile of the coupled system composed of honeycomb layers stacked along thezdirection. For each model system, we plot the layer-resolved wave function amplitudes along a particular direction in the momentum space and the 2D distribution of states localized along thezdirection. In each model, the Chern number distribution of the four bands on the top surface layer is indicated by a vectorC=[n1,n2,n3,n4]. In all cases except the case (b), the two high (low)-energy bands with the Chern numbern1,n2(n3,n4) are buried in the conduction (valence) band of the 3D NI. In the case of (b), the second band with the Chern numbern2=0 is in the gap. (a)C=[0,0,−1,+1]. (b)C=[−1,0,+1,0]. (c)C=[0,−1,+1,0]. (d)C=[−1,−1,+1,+1]. (e)C=[−1,+1,+1,−1]. In all cases, only the 2D bands with non-zero Chern numbers support bound states localized along thezdirection. Figure 5: Energy dispersion and distribution of localized states of 2D four-band QHI bulk bands in a continuum of the 3D NI. Energy dispersion and localization profile of the coupled system composed of honeycomb layers stacked along the z direction. For each model system, we plot the layer-resolved wave function amplitudes along a particular direction in the momentum space and the 2D distribution of states localized along the z direction. In each model, the Chern number distribution of the four bands on the top surface layer is indicated by a vector C =[ n 1 , n 2 , n 3 , n 4 ]. In all cases except the case ( b ), the two high (low)-energy bands with the Chern number n 1 , n 2 ( n 3 , n 4 ) are buried in the conduction (valence) band of the 3D NI. In the case of ( b ), the second band with the Chern number n 2 =0 is in the gap. ( a ) C =[0,0,−1,+1]. ( b ) C =[−1,0,+1,0]. ( c ) C =[0,−1,+1,0]. ( d ) C =[−1,−1,+1,+1]. ( e ) C =[−1,+1,+1,−1]. In all cases, only the 2D bands with non-zero Chern numbers support bound states localized along the z direction. Full size image Next, we describe the localization property of the 2D QHI with higher Chern number, in particular, when the Chern number of the conduction (valence) band is equal to −2 (+2). In this case, we expect that there should be at least two localized 2D bulk states in each of the valence or conduction band when each band is completely buried in a continuum. As shown in Fig. 6 , we can clearly see that there are several localized states that are well-separated in the momentum space. In particular, along the boundary of the Brillouin zone, it is numerically confirmed that there are three completely localized states. Among them, two states are related by the reflection symmetry but the other one is not. Therefore, there are at least two inequivalent localized states in the Brillouin zone, consistent with the prediction based on the consideration of topological invariants. 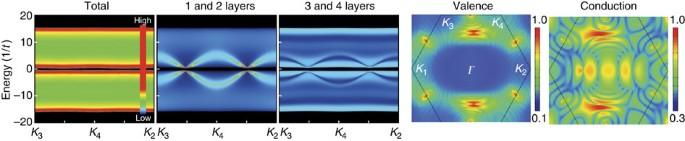Figure 6: Energy dispersion and distribution of localized states for the 2D QHI with Chern number two. Here the Chern numbers of the conduction and valence bands of the 2D QHI are −2 and +2, respectively. Notice that there are several localized bound states in the 2D Brillouin zone in both the valence and conduction bands of the 3D NI substrate as shown in the two panels on the right. On the left three panels, the dispersion of the coupled heterostructure, which is projected to the layers near the top surface of the system, is shown along the Brillouin zone boundary. Figure 6: Energy dispersion and distribution of localized states for the 2D QHI with Chern number two. Here the Chern numbers of the conduction and valence bands of the 2D QHI are −2 and +2, respectively. Notice that there are several localized bound states in the 2D Brillouin zone in both the valence and conduction bands of the 3D NI substrate as shown in the two panels on the right. On the left three panels, the dispersion of the coupled heterostructure, which is projected to the layers near the top surface of the system, is shown along the Brillouin zone boundary. Full size image Finally, let us consider the localization property of the 2D quantum spin Hall insulator on a substrate. As the quantum spin Hall insulator (QSHI) can be considered as a superposition of two QHI systems possessing opposite Chern numbers [11] , the topological protection of the bulk and edge states is expected to be observed in the QSHI heterostructure. As for the topological property of the QSHI, it is important to clarify whether the z component of the total spin, that is, S z , is conserved or not. When S z is conserved (not conserved), the topological invariant of the 2D system is the spin Chern number (the Z 2 invariant). In addition, we consider two different model Hamiltonians for the 3D NI. One is the two-band model breaking the time-reversal symmetry and the other is the four-band model preserving the time-reversal symmetry. In the case of the two-band model on the honeycomb lattice, as there is only one available state in each site, it can be considered as a spin-polarized system breaking the time-reversal symmetry. As shown in Fig. 7a , when the 3D NI breaks the time-reversal symmetry, several localized bound states are found independent of the presence ( Fig. 7a ) or absence ( Fig. 7b ) of the S z conservation. On the other hand, when the total heterostructure maintains the time-reversal symmetry, the S z conservation is crucial to obtain localized bound states. When the S z is conserved, several completely localized bound states appear as shown in Fig. 7c . However, surprisingly, once the S z conservation is violated owing to the Rashba-type spin-mixing term, all the 2D bulk states of the QSHI spread along the z direction, as shown in Fig. 7d . It is numerically confirmed that there is no localized bound state in the Brillouin zone. This observation demonstrates the fundamental difference between the Chern number (or spin Chern number) and the Z 2 invariant. In contrast to the case of the Chern number, the non-zero Z 2 invariant cannot protect any localized bound state in a continuum state. 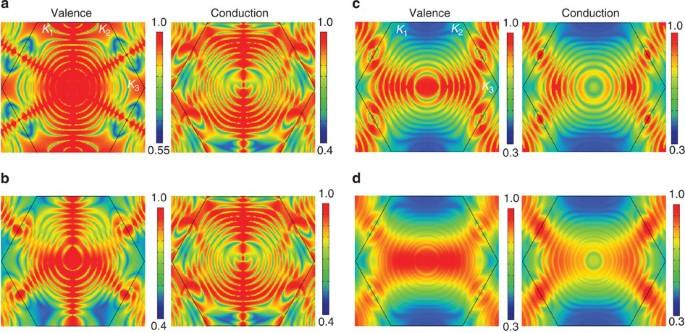Figure 7: The 2D distribution of localized states of the 2D QSHI bulk bands in 3D continuum states. (a,b) corresponds to the case when the 3D bulk breaks the time-reversal symmetry. In (c,d), the total system preserves the time-reversal symmetry. Thezcomponent of the total spin (Sz) is conserved in (a,c) whileSzis not conserved in (b,d) owing to the Rashba-type spin-mixing term. In all cases, the two high (low)-energy bands of the QSHI are buried in the conduction (valence) band continuum of the 3D NI. When the 3D bulk states break the time-reversal symmetry, there are localized bound states independent of theSzconservation (a,b). On the other hand, when the total system preserves the time-reversal symmetry, localized bound states exist whenSzis conserved (c) while all 2D states spread along thezdirection whenSzis not conserved (d). Figure 7: The 2D distribution of localized states of the 2D QSHI bulk bands in 3D continuum states. ( a , b ) corresponds to the case when the 3D bulk breaks the time-reversal symmetry. In ( c , d ), the total system preserves the time-reversal symmetry. The z component of the total spin ( S z ) is conserved in ( a , c ) while S z is not conserved in ( b , d ) owing to the Rashba-type spin-mixing term. In all cases, the two high (low)-energy bands of the QSHI are buried in the conduction (valence) band continuum of the 3D NI. When the 3D bulk states break the time-reversal symmetry, there are localized bound states independent of the S z conservation ( a , b ). On the other hand, when the total system preserves the time-reversal symmetry, localized bound states exist when S z is conserved ( c ) while all 2D states spread along the z direction when S z is not conserved ( d ). Full size image The existence of 2D bulk states localized along the z direction in a continuum protected by topology reveals the dual role played by the topological invariant. Conventionally, the topological invariant has been considered as a quantity that protects the extended bulk states against the localization owing to disorder. These extended bulk states protected by topology guarantee the existence of the delocalized states on the sample boundary even in the presence of disorder, which gives rise to the profound relationship between the bulk topological invariant and the extended boundary states, dubbed the bulk-boundary correspondence. For example, in integer quantum Hall systems, the Chern number can be formulated in terms of the number of chiral edge modes [21] , [22] , [23] . Also, the Z 2 invariants of 2D (3D) time-reversal invariant systems determine the parity of the number of helical edge modes (Dirac cones) at the boundary [24] . These boundary states within the bulk band gap smoothly connect the bulk valence and conduction bands, which can be deformed and fully merged into the bulk bands only when the corresponding bulk topological invariant changes through the bulk band gap closing. Namely, the pair annihilation of the topological invariants is the only mechanism to eliminate the extended states. On the other hand, when the topological insulator is coupled to a substrate material, the topological invariant also guarantees the existence of some bulk states localized along the z direction, which are effectively decoupled from the continuum states of the substrate. In the case of the 2D QHI on a topologically trivial 3D NI, the Chern number of the QHI determines the minimum number of localized 2D QHI bulk states buried in the continuum states of the 3D NI. The essential ingredient leading to the localized 2D bulk states buried in a continuum is the inequivalence of the Chern numbers between the 2D QHI and the effective 2D system constituting the 3D NI. Therefore, if the topological property of the QHI on the top layer can be controlled by tuning the bulk band gap of the 2D QHI, the completely localized states can start to be hybridized with the continuum states of the 3D NI across the topological phase transition and be spread through the whole sample in the end when the 2D bulk state on the top layer is deep inside of the topologically trivial phase. In addition, using the same framework, it is also possible to understand the evolution of the energy band structure of the coupled 2D QHI systems stacked along the vertical z direction. Here, we assume that the inter-layer coupling is not so strong to induce any band touching through the inter-layer hybridization. If we distinguish the QHI on the top layer from the other part of the system, the whole system can be considered as a heterostructure composed of a 2D QHI layer and a 3D QHI substrate. As the top layer and the effective 2D layer of the 3D substrate have the same Chern number, there can be no 2D bulk state that is localized on the top layer, which is confirmed through the additional numerical study discussed in detail in Supplementary Note 5 with figures shown in Supplementary Fig. S2 . In this case, the 1D CESs of the top QHI layer should also be delocalized and spread along the vertical z direction. The extended 1D CESs eventually participate in the formation of the boundary gapless states of the 3D weak QHI [25] , which disperse along the two orthogonal directions, one of which corresponds to the vertical z direction [26] . To establish the general relationship between the topological invariant of the 3D substrate and the localization property of the 2D QHI is an interesting problem requiring additional studies. Let us briefly discuss the influence of disorder. As shown above, the bound states exponentially localized along z direction exist only at several discrete k -points. As the disorder scattering mixes the wavefunctions at different k -points, it is expected that the bound states can be hybridized with extended states and hence delocalized along the z direction. Correspondingly, the delta-functional peak of the spectral function will turn into a broadened resonance. The edge channels, on the other hand, can be protected by the gap, and hence remain localized along the z direction. However, these hand-waving arguments should be confirmed by more careful analysis, which is left for future studies. We conclude with a discussion of candidate materials realizing the topological protection of localization. A recent LDA+U study has proposed that several pyrochlore iridates can be anti-ferromagnetic insulators with the all-in/all-out spin configuration [27] . In this magnetic state, the [111] surface or any of its symmetry equivalents supports a kagome-lattice plane with a non-coplanar spin ordering. As the spin chirality induced by non-coplanar spins can give rise to a QHI on the surface [28] while the bulk insulating state is topologically trivial, pyrochlore iridates are an ideal platform to realize intriguing localization phenomena protected by topology. Lattice Hamiltonian of the stacked 2D honeycomb lattice system In each honeycomb layer, in addition to the hopping amplitude t between nearest-neighbour sites, we take into account of two additional terms, that is, the staggered chemical potential μ s between two sublattice sites in a unit cell and the imaginary hopping amplitude λ so between next nearest-neighbour sites. Explicitly, the Hamiltonian including μ s and λ so can be written as where are Pauli matrices indicating the two sublattice sites and , . In this Hamiltonian, when ( ), the system is a QHI (a trivial insulator) [4] . Here, we take \(H_{\mu _s = 0,\lambda so} \) as a model Hamiltonian for QHI. Also, we use \(H_{\mu _s ,\lambda so = 0} \) as a basis to construct a 3D NI by incorporating inter-layer hopping amplitudes. Then the Hamiltonian for the coupled system can be written as where and .For numerical computation, we choose λ so =1, T 0 =3, T z =0.3. t=1 ( t=3.5 ) for ( ). To control the energy gap of 3D NI, we use μ s =20 for Fig. 2a , μ s =12 for Fig. 2b and μ s =7.5 for Fig. 2c . For the construction of general lattice models, we replace the basis for the 3D NI by the following Hamiltonian, where t′ is the hopping amplitude between next nearest-neighbour sites. Here, the hybridization between two sublattice sites μ′ determines the size of the band gap. The Hamiltonian for a 3D NI can be obtained by stacking H NNN along the z direction. Existence of 1D CES under hybridization The influence of the coupling to the 3D continuum states on the existence of the 1D CESs can be considered in the following way. We first consider a decoupled 2D QHI described by the Green’s function where x ( k y ) is the spatial (momentum) coordinate and is the energy. Let V ( x 0 ) be a local perturbation creating a boundary at x = x 0 parallel to the y direction. Then the system with a boundary can be described by the Green’s function which satisfies the equation where the k y coordinate is omitted [29] . After simple algebra, we can show that which leads to the following condition to obtain the edge state Now, we turn on the coupling to the 3D continuum state under which promotes to satisfying , the retarded Green’s function in equation (1). Considering the local potential V ( x 0 ) again, the condition to obtain an edge state can be derived simply by replacing by G QHI in equation (3). The point is that when is within the bulk gap of 3D substrate because develops the imaginary part only when is within the 3D continuum states. Therefore, the coupling to 3D continuum states does not affect the existence of edge states. Moreover, in the case of the zero-energy edge state, the condition to obtain the in-gap state can be rewritten in terms of the thermal Green’s function at zero Matsubara frequency . Namely, determines the condition to obtain the zero-energy in-gap state. It is interesting to note the consistency of this result with the recent work proposing that the topological invariant of general interacting systems can be written in terms of the Green’s function at zero Matsubara frequency [30] . How to cite this article: Yang, B.-J. et al. Topological protection of bound states against the hybridization. Nat. Commun. 4:1524 doi: 10.1038/ncomms2524 (2013).